UV-B irradiation-activated E3 ligase GmILPA1 modulates gibberellin catabolism to increase plant height in soybean 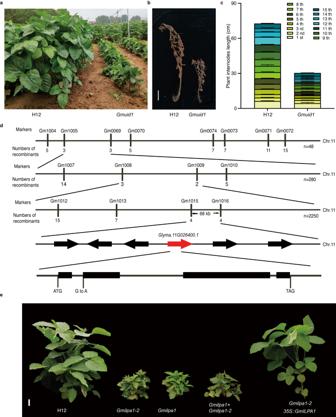Fig. 1: Identification and characterization of the dwarf mutantGmuid1. aRepresentative image of plants from the wild-type (WT) Hedou 12 (H12) and theGmuid1mutant at the vegetative stage in the field.bRepresentative images of the WT andGmuid1at the R8 stage (full maturity). Scale bar, 10 cm.cInternode length of WT andGmuid1plants at the R8 stage. Data are means ± standard deviation (SD),n= 6 independent plants.dSummary of the positional cloning of theGmUID1(also namedGmILPA1) locus to chromosome 11. The insertion/deletion (InDel) markers Gm1005 and Gm0069 were used for initial mapping.GmUID1(GmILPA1) was fine-mapped to a 68-kb region between the single sequence repeat (SSR) markers Gm1015 and Gm1016 on chromosome 11.nrepresents individual F2/F3plants with the mutant phenotype.eRepresentative images of H12,Gmilpa1-2(Gmuid1),Gmilpa1,Gmilpa1-2×Gmilpa1F1, andGmilpa1-2 35S:GmILPA1plants at the R1 stage (beginning of flowering). Scale bar, 10 cm. Source data are provided as a Source Data file. Plant height is a key agronomic trait that affects yield and is controlled by both phytohormone gibberellin (GA) and ultraviolet-B (UV-B) irradiation. However, whether and how plant height is modulated by UV-B-mediated changes in GA metabolism are not well understood. It has not been reported that the E3 ubiquitin ligase Anaphase Promoting Complex/Cyclosome (APC/C) is involved in the regulation of plant growth in response to environmental factors. We perform a forward genetic screen in soybean and find that a mutation in Glycine max Increased Leaf Petiole Angle1 ( GmILPA1 ), encoding a subunit of the APC/C, lead to dwarfism under UV-B irradiation. UV-B promotes the accumulation of GmILPA1, which ubiquitinate the GA catabolic enzyme GA2 OXIDASE-like (GmGA2ox-like), resulting in its degradation in a UV-B-dependent manner. Another E3 ligase, GmUBL1, also ubiquitinate GmGA2ox-like and enhance the GmILPA1-mediated degradation of GmGA2ox-like, which suggest that GmILPA1-GmGA2ox-like module counteract the UV-B-mediated reduction of bioactive GAs. We also determine that GmILPA1 is a target of selection during soybean domestication and breeding. The deletion (Indel-665) in the promoter might facilitate the adaptation of soybean to high UV-B irradiation. This study indicates that an evolutionary GmILPA1 variant has the capability to develop ideal plant architecture with soybean cultivars. Ideotype breeding aims to achieve high yields in crops by combining multiple beneficial genetic traits into one variety. Plant height is an important feature of plant ideotypes. The application of semi dwarf varieties has significantly improved crop yield by increasing the planting density and the lodging resistance [1] , [2] . The gains in grain productivity during the Green Revolution were a direct consequence of optimal plant height [3] . Mutant alleles of the Green Revolution genes Semidwarf1 ( Sd1 ) and Reduced height ( Rht ) are utilized to improve crop yields by decreasing overall plant height and increasing the harvest index [4] . Although dozens of quantitative trait loci (QTLs) have been identified that control plant height in soybean ( Glycine max L.), few of the causal genes have been isolated and characterized [5] , [6] . For example, GmDW1 ( DWARF 1 ) encodes an ent-kaurene synthase [7] , GmLHY ( LATE ELONGATED HYPOCOTYL ) encodes an MYB transcription factor, Determinate stem 1 ( Dt1 ) is a homolog of TERMINAL FLOWER 1 , and Dt2 encodes dominant MADS domain factor [8] , [9] , [10] could help deploy the semi-dwarf phenotype and improve soybean yields. The plant hormone gibberellins play a pivotal role in determining plant height [11] , [12] . Mutations in genes involved in GA biosynthesis, metabolism, and signaling influence plant height. Key components of the GA signaling pathway have been identified from genetic screens performed in rice ( Oryza sativa ) and Arabidopsis ( Arabidopsis thaliana ). For instance, DELLA proteins restrain plant growth, and their degradation upon perception of GA signal promotes growth [13] . Loss-of-function mutations in GA biosynthetic genes such as GA20ox and GA3ox lead to dwarfism [14] , [15] , [16] , [17] , [18] , [19] . Conversely, GA2ox members are GA catabolic enzymes that inactivate the phytohormone and negatively regulate plant growth, and the overexpression of their encoding genes suppresses stem growth [20] , [21] , [22] , [23] , [24] . Several transcription factors can also negatively regulate GA-mediated stem cell elongation by activating GA2ox transcription [25] , [26] . Furthermore, GA2ox expression is induced by environmental signals, including salt stress, high temperature, and light [27] , [28] , [29] , [30] . While much is known about the transcriptional modulation of GA2ox s, whether and how GA2oxs are post-translationally regulated are largely unknown. Exposure to ultraviolet-B (UV-B) light is an abiotic stressor that affects plant height [31] , [32] . In Arabidopsis , inhibition of hypocotyl growth involves the transcriptional activation of ELONGATED HYPOCOTYL5 ( HY5 ) and HY5 HOMOLOG ( HYH ) by the UV-B photoreceptor UV RESISTANCE LOCUS8 (UVR8), HY5/HYH stability, and the degradation of the transcription factors PHYTOCHROME-INTERACTING FACTOR4 (PIF4) and PIF5 [32] , [33] , [34] , [35] . In addition, UV-B also inhibits plant growth in Arabidopsis by promoting the accumulation of DELLA proteins, thus repressing GA signaling output [36] . UV-B exposure also decreases the transcript levels of GA biosynthesis genes, such as GA3ox and GA20ox , and increases the transcript levels of GA2ox [37] to inhibit hypocotyl growth. To date, UV-B has only been shown to affect the transcription of GA biosynthesis and catabolism genes. The ubiquitin-proteasome system (UPS) is a major regulatory mechanism for the selective degradation of proteins in eukaryotes [38] and plays a key role in plant growth and development [39] , [40] , [41] , [42] , [43] . Ubiquitin is attached to substrate proteins by a series of enzymatic reactions. First, ubiquitin molecules are activated by an E1 activating enzyme in an ATP-dependent manner, followed by its transfer to an E2 conjugating enzyme, and finally covalent attachment to the target protein by an E3 ubiquitin ligase [44] . Ubiquitin tags label target proteins for degradation via the 26S proteasome using its ATP-dependent endopeptidase activity [45] . Each E3 ubiquitin ligase strictly controls the efficiency and substrate specificity of the UPS. E3 ubiquitin ligases are divided into four types: HECT (Homology to E6AP C Terminus), RING/U-box (Really Interesting New Gene/U-Box), SCF (Skp1, Cullin, and F-box protein complex), and APC/C (anaphase promoting complex/cyclosome) [46] . Of these, the APC/C is a conserved multi-subunit ubiquitin ligase assembled from 13 different subunits and plays an important role during the cell cycle [47] . The APC/C is also involved in plant growth and development, modulating plant height, leaf size, lateral root number, and silique development [48] . In addition, APC/C activity was reported to influence phytohormone signals, as auxin distribution is disrupted in embryos of apc4 mutants [49] . In rice, the apc6 mutant has a shorter stature and does not respond to exogenous GA [50] . However, APC/C-mediated regulation of plant growth and development by environmental factors has not been reported. In this study, we identified a soybean dwarf mutant in a forward genetic screen. The Gmuid1 (soybean UV-B induced dwarfism1 ) mutant showed a dwarf phenotype in a UV-B-dependent manner. And we found that the mutation in Glycine max Increased Leaf Petiole Angle1 ( GmILPA1 ), encoding an APC8-like protein, resulted in the dwarfism of Gmuid1 under UV-B irradiation. We further demonstrated that UV-B induces the accumulation of GmILPA1, which reduced UV-B-induced growth inhibition by interacting with GmGA2ox-like and targeting it for degradation in response to UV-B. Another E3 ubiquitin ligase, GmUBL1, interacted with both GmILPA1 and GmGA2ox-like, respectively, to promote degradation of GmGA2ox-like. Our findings indicated that GmILPA1 promotes GA catabolism to modulate plant height under UV-B exposure. Our study characterized the effect of UV-B exposure and GA application on plant height, with a view to gain a better understanding of the mechanism of APC/C by UV-B-mediated dwarfism in soybean. Importantly, GmILPA1 underwent artificial selection during soybean domestication, with the four major haplotypes GmILPA1 Hap1 , GmILPA1 Hap2 , GmILPA1 Hap5 and GmILPA1 Hap6 having been targeted by selection in improved cultivars. The shorter height of plants harboring GmILPA1 Hap5 might be due to the specific mutations in cis-regulatory elements affecting the response to UV-B. GmILPA1 is a positive regulator of plant height in soybean To isolate novel genes that regulate plant height in soybean, we performed a forward genetic screen of the Chinese soybean cultivar Hedou 12 (H12) mutagenized with ethyl-methanesulfonate (EMS). We identified the mutant Gmuid1 in M4 populations based on its shorter plant height and internode length when grown in the field compared to H12 plants (Fig. 1a–c ). Gmuid1 plants also had smaller leaves, shorter petioles, and a larger leaf petiole angle than in H12 (Supplementary Fig. 1a, b ). We investigated the underlying cellular basis of the short internodes of Gmuid1 by measuring cell length in Gmuid1 and H12 plants. Compared to H12, longitudinal parenchyma cells in Gmuid1 internodes were significantly shorter (Supplementary Fig. 1c, d ). Furthermore, we observed no significant difference in the number of nodes along the main stem and branches between H12 and Gmuid1 ; however, the other agronomic traits, including number of pods, number of seeds per plant, grain weight per plant, and hundred-grain weight, were all lower in Gmuid1 than in H12 (Supplementary Fig. 1e–j ). Fig. 1: Identification and characterization of the dwarf mutant Gmuid1 . a Representative image of plants from the wild-type (WT) Hedou 12 (H12) and the Gmuid1 mutant at the vegetative stage in the field. b Representative images of the WT and Gmuid1 at the R8 stage (full maturity). Scale bar, 10 cm. c Internode length of WT and Gmuid1 plants at the R8 stage. Data are means ± standard deviation (SD), n = 6 independent plants. d Summary of the positional cloning of the GmUID1 (also named GmILPA1 ) locus to chromosome 11. The insertion/deletion (InDel) markers Gm1005 and Gm0069 were used for initial mapping. GmUID1 ( GmILPA1 ) was fine-mapped to a 68-kb region between the single sequence repeat (SSR) markers Gm1015 and Gm1016 on chromosome 11. n represents individual F 2 /F 3 plants with the mutant phenotype. e Representative images of H12, Gmilpa1-2 ( Gmuid1 ), Gmilpa1 , Gmilpa1-2 × Gmilpa1 F1, and Gmilpa1-2 35S:GmILPA1 plants at the R1 stage (beginning of flowering). Scale bar, 10 cm. Source data are provided as a Source Data file. Full size image To identify the causative gene responsible for the observed phenotypic changes, we crossed the soybean cultivar Williams 82 to the Gmuid1 mutant, yielding an F 2 population comprising 201 individual F 2 plants. Of these F 2 plants, 153 showed the wild-type phenotype and 48 exhibited the mutant phenotype, thus fitting a 3:1 segregation ratio ( χ 2 test, P = 0.89). This result indicated that the Gmuid1 mutation affects a single gene and is recessive. We used 128 INDEL markers and the 48 individual F 2 plants to map the GmUID1 locus, the results indicated that the mutant locus was mapped to a 4.5-Mb genomic region between markers Gm1005 and Gm0069 on chromosome 11, based on the soybean reference genome from Williams 82 [51] . We then developed new molecular markers within this interval and genotyped a set of 280 individual F 2 plants with the mutant phenotype from new F 1 inbred offspring, which allowed us to narrow down the interval to a 0.72-Mb region between INDEL markers Gm1008 and Gm1009. We further developed F 3 lines from F 2 lines homozygous for the Gmuid1 mutation but heterozygous at one of the flanking markers, culminating in a 68-kb region between SSR markers Gm1015 and Gm1016 based on 2250 F 2 and F 3 individuals. This interval contains six open reading frames in the Williams 82 reference genome [51] (Fig. 1d ). Independently, we performed a bulk segregant analysis using two sets of pooled F 2 plants exhibiting the mutant or wild-type (WT) phenotype (a mix of homozygous and heterozygous plants for the WT allele) to identify all single nucleotide polymorphisms (SNPs) relative to Williams 82 and calculate the SNP index for each pool. The sequencing depth of each pool was 40× genome coverage. This analysis highlighted a region near the top of chromosome 11 (Supplementary Fig. 2a-b ), which was consistent with the map-based cloning above. Importantly, we identified one SNP (G-to-A at position 222 of genomic DNA) in the splicing site of the first intron for candidate gene Glyma.11G026400.1 in the Gmuid1 mutant; the remaining five candidate genes showed no SNPs between H12 and Williams 82 (Fig. 1d ). The single nucleotide substitution at the splicing site altered messenger RNA (mRNA) splicing and led to premature termination in the new increased exon of the transcript encoded by Glyma.11G026400 in the Gmuid1 mutant (Supplementary Fig. 3 ). Therefore, we identified a candidate gene for regulating plant height. Additionally, Glyma.11G026400 was previously reported and named GmILPA1 ( Glycine max Increased Leaf Petiole Angle1 ) [52] ; the mutant Gmilpa1 resulted in the deletion of exon 4 of Glyma.11G026400 [52] , [53] (Supplementary Fig. 4a ). Similar to Gmuid1 , the Gmilpa1 mutant also showed a dwarf phenotype in the field (Fig. 1e , Supplementary Fig. 4b ). As expected, F 1 plants from the cross between Gmuid1 and Gmilpa1 also exhibited the dwarf phenotype (Fig. 1e , Supplementary Fig. 4c, d ). Therefore, Gmuid1 is an allelic mutant of Gmilpa1 , we renamed the Gmuid1 as Gmilpa1-2 . In addition, we obtained transgenic lines overexpressing its coding sequence cloned in-frame with that of the green fluorescent protein gene ( GFP ) in the Gmilpa1-2 mutant background. We obtained six independent transformation events; their T 2 progeny accumulated GFP and restored the mutant phenotype to the WT, as evidenced by plant height (Fig. 1e and Supplementary Fig. 4e–f ). Collectively, all these results indicated that Glyma.11G026400 is GmUID1 ( GmILPA1 ), which controls plant height in soybean. Sequence comparison and phylogenetic analysis demonstrated that GmILPA1 encodes an APC8-like protein, a subunit of the APC/C (Supplementary Fig. 5a ). Reverse transcription quantitative PCR (RT-qPCR) analysis indicated that GmILPA1 is constitutively expressed in roots, hypocotyls, cotyledons, stems, leaves, flowers, and pods (Supplementary Fig. 5b ). We also transiently expressed a GmILPA1-GFP fusion construct driven by the cauliflower mosaic virus (CaMV) 35S promoter in Nicotiana benthamiana leaves, in agreement with previous report [53] , we also found that GmILPA1-GFP localizes to both the nucleus and cytoplasm (Supplementary Fig. 5c ). GmILPA1 promotes plant height in a UV-B-dependent manner To further characterize the Gmilpa1-2 mutant, we performed phenotypic analyses in a glasshouse. To our surprise, Gmilpa1-2 plants did not have a dwarf phenotype under these conditions (Fig. 2a, b ). Considering the differences between the light spectra of sunlight and white light-emitting diodes (LEDs) [54] , we hypothesized that the differential phenotype of Gmilpa1-2 might be caused by the lack of UV-B light from LEDs. To test this hypothesis, we grew H12, Gmilpa1-2 and Gmilpa1 seedlings under white light (600 μmol m –2 s –1 white light, no UV-B, 25 °C, and a 12-h-light/12-h-dark photoperiod) and white light supplemented with UV-B (600 μmol m –2 s –1 white light, 1.5 μmol m −2 s −1 UV-B, 25 °C, and a 12-h-light/12-h-dark photoperiod) to the V2 stage. We observed shorter plants with Gmilpa1-2 and Gmilpa1 relative to H12 in response to UV-B irradiation (Fig. 2c, d ). We concluded that UV-B is essential for evoking the dwarf phenotype of the Gmilpa1 mutant. Fig. 2: UV-B is required for the Gmilpa1-2 phenotype. a Representative image of the WT Hedou 12 (H12) and Gmilpa1-2 grown in a glasshouse at the V4 stage (four unrolled trifoliate leaves). Scale bar, 10 cm. b Height of the plants shown in ( a ), ( n = 7 biologically independent samples; P = 0.1909), P- values were calculated by comparing to H12 plants using two-tailed Student’s t -test; ns not significant. c Representative images of the V2 stage of H12, Gmilpa1-2 , and Gmilpa1 grown under white light (600 μmol m –2 s –1 white light, no UV-B, 25 °C, and a 12-h-light/12-h-dark photoperiod) and white light supplemented with UV-B (600 μmol m –2 s –1 white light, 1.5 μmol m −2 s −1 UV-B, 25 °C, and a 12-h-light/12-h-dark photoperiod). Scale bar, 10 cm. d Height of the seedlings shown in ( c ), ( n > 6 biologically independent samples; P = 2.42 × 10 −6 in H12 and Gmilpa1-2 , P = 1.80 × 10 −6 in H12 and Gmilpa1 ). Data are presented as mean values ± SD; P- value is calculated with a one-way ANOVA analysis–Tukey comparison, and the columns labeled without the same alphabet are significantly different ( P < 0.05, two-sided). *** P < 0.001, ns not significant. Source data are provided as a Source Data file. Full size image UV-B promotes the interaction between GmILPA1 and GmGA2ox-like To investigate how GmILPA1 regulates plant height in soybean, we performed a yeast two-hybrid (Y2H) screen with a soybean cDNA library to identify GmILPA1-interacting proteins. Among the potential candidate interactors, we noticed two proteins with potential roles in modulating plant height. Indeed, one positive clone encodes 2-oxoglutarate–dependent dioxygenase (2ODD), which is a close homolog of Arabidopsis GA2ox4 that we named GmGA2ox-like (Supplementary Fig. 6a ). To confirm GmGA2ox-like is a functional GA2-oxidase, we performed the in vitro enzymatic activity assay using GA 1 and GA 4 as the substrates. The results showed that GmGA2ox-like converted GA 1 and GA 4 to their corresponding 2β-hydroxylated products GA 8 and GA 34 , respectively (Supplementary Fig. 6b, c ). Next, we generated 3 lines overexpressing GmGA2ox-like , which displayed a dwarf phenotype compared to non-transgenic WT plants (Supplementary Fig. 6d, e ). Sequence analysis revealed that GmGA2ox-like harbors a typical D-box (Supplementary Fig. 6f ). The second clone encodes a protein with a RING/U-box domain that is predicted to have E3 ubiquitin ligase activity; we named this protein GmUBL1 (ubiquitin ligase 1). To validate these interactions, we carried out yeast two-hybrid (Y2H) assays. The Y2H assay showed that GmILPA1 interacts with GmGA2ox-like and GmUBL1, respectively (Fig. 3a ). To confirm these interactions in vivo, we performed bimolecular fluorescence complementation (BiFC) and co-immunoprecipitation (Co-IP) assays in N. benthamiana leaves transiently expressing the appropriate pairs of constructs. We detected yellow fluorescence protein (YFP) fluorescence signals in N. benthamiana epidermal cells co-expressing GmILPA1-YFP C (encoding a fusion between GmILPA1 and the C-terminal half of YFP) and GmGA2ox-like-YFP N (encoding a fusion between GmGA2ox-like and the N-terminal half of YFP) or GmILPA1-YFP C and GmUBL1-YFP N (Fig. 3b ). We also confirmed these protein interactions by Co-IP assays as well (Fig. 3c, d , Supplementary Fig. 7c ). We asked whether GmGA2ox-like and GmUBL1 might also interact. We explored this possibility with Y2H, BiFC, and Co-IP assays. Indeed, we determined that GmGA2ox-like also interacts with GmUBL1 with all three assays (Fig. 3a, b, e ). Together, our results demonstrated that GmILPA1, GmGA2ox-like, and GmUBL1 interact with each other. In addition, GmILPA1 and GmGA2ox-like, and GmILPA1 and GmUBL1 were co-localized, respectively, in the cytoplasm and nucleus by transient expression in N. benthamiana leaves (Supplementary Fig. 8a, b ). Fig. 3: GmILPA1 interacts with GmGA2ox-like and GmUBL1. a Yeast two-hybrid assays showing the interactions among GmILPA1, GmGA2ox-like, and GmUBL1. GmILPA1 and GmUBL1 were fused to GAL4-BD, and GmGA2ox-like was fused to GAL4-AD when encoded by the pGADT7 and pGBKT7 vectors. Serial dilutions of equivalent amounts of yeast were plated on synthetic defined (SD) medium without Leu (L), Trp (T) (SD-L-T), or without Leu (L), Trp (T), and His (H) (SD-L-T-H) containing 1 mM 3-amino-1,2,4-triazole (3-AT), with growth on triple dropout media indicating an interaction between the tested proteins. b A BiFC assay used to verify the interactions among GmILPA1, GmGA2ox-like, and GmUBL1 in vivo in N. benthamiana leaves. The non-interacting proteins, mGmGA2ox-like (mutated construct of D-Box motif) and GmPUB21 (a U-Box E3 Ubiquitin Ligases), were used as a negative control. Scale bars, 50 μm. c – e Co-IP of GmILPA1, GmGA2ox-like, and GmUBL1. Immunoprecipitation was performed with anti-GFP-agarose beads using N. benthamiana leaves co-infiltrated with the constructs GmGA2ox-like-GFP and GmILPA1-MYC ( c ), GmUBL1-GFP and GmILPA1-MYC ( d ), or GmUBL1-GFP and GmGA2ox-like-MYC ( e ). f BiFC assays indicating that UV-B treatment promotes the interaction between GmILPA1 and GmGA2ox-like. N. benthamiana leaves were co-infiltrated with GmGA2ox-like–nYFP and GmILPA1–cYFP and exposed to 1 h of UV-B (21 μmol m −2 s −1 ) or kept in white light before imaging. Scale bars, 50 μm. g Relative YFP fluorescence intensity in the cytoplasm from the images in ( f ), ( n = 30 cells, P = 1.30 × 10 −5 ), the relative fluorescence intensities of cytoplasm and whole cells were quantified and the cytoplasm-to- background ratios are plotted. Data are presented as mean values ± SD, Student’s t -test was used for the significance test, *** P < 0.001. h Co-IP assays showed that UV-B increased the interaction between GmILPA1 and GmGA2ox-like. N. benthamiana were co-transformed with GmGA2ox-like-GFP and GmILPA1-MYC , and treated with or without 12 h UV-B. Then, they were used in the co-immunoprecipitation assay. Immunoprecipitation was performed using GFP-Trap agarose beads, and the immunoblots were probed using anti-myc and anti-GFP antibodies. Source data are provided as a Source Data file. Full size image As Gmilpa1-2 showed a dwarf phenotype only upon UV-B exposure, we investigated the potential effect of UV-B on the interaction between GmILPA1, GmGA2ox-like, and GmUBL1. BiFC assays indicated that UV-B treatment promotes the interaction between GmILPA1 and GmGA2ox-like in the cytoplasm, as evidenced by the three-fold higher relative fluorescence intensity detected in the cytoplasm following treatment with UV-B relative to controls maintained under white light throughout (Fig. 3f, g ). We further tested the effect of UV-B on the interaction of GmILPA1 and GmGA2ox-like using Co-IP assays. The result showed that UV-B enhanced the interaction between GmILPA1 and GmGA2ox-like (Fig. 3h ). However, UV-B treatment failed to affect the interaction between GmILPA1 and GmUBL1 or between GmGA2ox-like and GmUBL1 (Supplementary Fig. 7d–i ). These results demonstrated that UV-B light promotes the interaction between GmILPA1 and GmGA2ox-like. GmILPA1 mediates the degradation of GmGA2ox-like in a UV-B-dependent manner The APC/C facilitates the ubiquitination and subsequent degradation of specific proteins by the UPS, raising the possibility that GmGA2ox-like might be targeted for degradation by GmILPA1. To test this hypothesis, we co-expressed constructs encoding N-terminally FLAG-tagged ubiquitin (FLAG-Ub) and C-terminally GFP-tagged GmGA2ox-like (GmGA2ox-like-GFP) in N. benthamiana leaves via Agrobacterium ( Agrobacterium tumefaciens )–mediated transient expression, followed by Co-IP with anti-GFP antibodies. We detected a smear representing poly-ubiquitinated GmGA2ox-like by immunoblotting with an anti-FLAG antibody (Fig. 4a ), indicating that GmGA2ox-like is indeed subjected to polyubiquitination in plant cells. We then used a bioinformatics web tool to identify amino acids in GmGA2ox-like that are modified by ubiquitination, yielding the residues K394 and K407. We replaced each lysine residue by arginine (K394R, K407R, and K394R K2407R) and transiently expressed constructs encoding GmGA2ox-like-GFP harboring one or both mutations in N. benthamiana leaves to assess their effect on protein stability and ubiquitination. Accordingly, we immunoprecipitated total protein extracts with anti-GFP antibodies, followed by immunoblot analysis with anti-Ub antibodies. We observed smears in the immunoblots for intact GmGAox2-like and the K407R variant, but did not detect smears for the K394R or K394R K407R variant (Fig. 4b ) which may indicate that K394 is the key residue for GmILPA1 ubiquitination. Fig. 4: GmGA2ox-like is ubiquitinated and degraded by the proteasome. a In vivo ubiquitination of GmGA2ox-like as detected by co-immunoprecipitation (Co-IP) assay. b Identification of the ubiquitination sites essential for GmGA2ox-like ubiquitination. c Ubiquitination of GmGA2ox-like by GmILPA1 in vitro. Brackets denote the ubiquitinated bands. d , e Ubiquitination of GmGA2ox-like by GmILPA1 in N. benthamiana leaves via Agrobacterium -mediated transient expression. f GmGA2ox-like is ubiquitinated in plants. Ubiquitinated proteins were enriched from the P62-agarose matrix that was incubated with total proteins isolated from three independent transgenic plants stably expressing GmGA2ox-like-GFP or from H12 plants. g Regulation of GmGA2ox-like stability by GmILPA1 in vivo. H12 and Gmilpa1-2 seedlings grown under white light and white light supplemented with UV-B to the V2 stage, and GmGA2ox-like was checked with an anti-GmGA2ox-like antibody. The band intensities in western blots were quantified ( h ), Data are presented as mean values ± SEM, n = 3 independent experiments. i Immunoblots showing GmGA2ox-like protein levels in V2 stage seedlings of H12 and Gmilpa1-2 grown in white light (600 μmol m −2 s −1 , 12 h/12 h light/dark) and then transferred to white light supplemented with UV-B (1.5 μmol m −2 s −1 , 12 h/12 h light/dark) for the indicated time periods. GmGA2ox-like abundance was detected with anti-GmGA2ox-like antibody and quantified ( k , l ). Data are presented as mean values ± SEM, n = 3 independent experiments. j GmGA2ox-like degradation in cell-free degradation assays in the presence of GmILPA1 and GmUBL1. GmGA2ox-like-MYC , GmUBL1-GFP , and GmILPA1-FLAG were individually infiltrated in N. benthamiana . GmGA2ox-like-MYC protein extracts were individually mixed with recombinant GmUBL1-GFP , GmILPA1-FLAG, GmUBL1-GFP , or GmILPA1-FLAG . Samples were collected at the indicated time points, and GmGA2ox-like abundance was probed by immunoblotting with anti-MYC antibody and quantified ( m ). Data are presented as mean values ± SEM, n = 3 independent experiments. Source data are provided as a Source Data file. Full size image To investigate whether GmILPA1 facilitates GmGA2ox-like degradation directly via ubiquitination, we performed in vitro ubiquitination assays. To this end, we used in vitro APC/C-ubiquitination assays, in which the APC/C complex (E3) immunoprecipitated from GmILPA1-GFP transgenic plants was incubated with Ub, ATP, E1, E2, and recombinant MBP-GmGA2ox-like. Our results showed that the E3 ligase GmILPA1 was auto-ubiquitinated as detected using the anti-Flag antibody (Fig. 4c ). Indeed, GmILPA1 promoted the ubiquitination of GmGA2ox-like in vitro, as evidenced by the smear for GmGA2ox-like-MBP in immunoblots using anti-MBP antibodies; however, GmGA2ox-like K394R cannot be ubiquitinated (Fig. 4c ). We co-expressed the GmGA2ox-like-GFP and GmILPA1-MYC in N. benthamiana leaves, followed by Co-IP with anti-myc antibodies and immunoblotting with anti-ubiquitin antibodies. We detected a remarkably increased smear signal representing poly-ubiquitinated GmGA2ox-like in the presence of GmILPA1 (Fig. 4d ). In addition, we used the same method to show that there was no remarkably increased smear signal of mGmGA2ox-like (mutated construct of D-Box motif) in the presence of GmILPA1 (Supplementary Fig. 9a ). We interpreted this result as evidence that GmGA2ox-like can be ubiquitinated by GmILPA1. As GmUBL1 has potential E3 ubiquitin ligase activity, we wondered if GmUBL1 might facilitate ubiquitination of GmGA2ox-like. We co-expressed the GmGA2ox-like-GFP and GmUBL1-MYC constructs in N. benthamiana leaves, followed by Co-IP with anti-myc antibodies and immunoblotting with anti-ubiquitin antibodies. Similarly, we detected a remarkably increased smear representing poly-ubiquitinated GmGA2ox-like in the presence of GmUBL1 (Fig. 4e ). This result showed that GmGA2ox-like can be ubiquitinated by GmUBL1. To determine whether GmGA2ox-like can be ubiquitinated in soybean, we used a P62-agarose matrix that is capable of binding ubiquitinated proteins to enrich the ubiquitinated proteins from three independent transgenic seedlings stably expressing 35S:GmGA2ox-like-GFP or from wild-type plants as a negative control. The bound proteins were used for immunoblotting analysis with anti-GFP antibody. The ladder-like protein pattern was detected in the enriched proteins from three transgenic plants but not from WT plants (Fig. 4f ). This result indicated that GmGA2ox-like can be ubiquitinated in soybean plants. To understand how GmILPA1 regulates the protein stability of GmGA2ox-like in soybean plants, we examined the GmGA2ox-like protein levels by western blotting with anti-GA2ox-like antibody (see Supplementary Fig. 7b for GmGA2ox-like antibody specificity) in WT and Gmilpa1-2 plants under both white light and white light supplemented with UV-B (600 μmol m –2 s –1 white light, 1.5 μmol m −2 s −1 UV-B, 25 °C, and a 12-h-light/12-h-dark photoperiod). We found lower levels of GmGA2ox-like under the white light supplemented with UV-B compared with that under the white light in the WT. In contrast, the GmGA2ox-like protein level was not reduced under the same conditions in the Gmilpa1-2 plants (Fig. 4g, h ). Moreover, V2 stage-grown WT and Gmilpa1-2 mutant seedings under white light were transferred to white light supplemented with UV-B or continued to grow under white light for the indicated time periods, and our immunoblot data showed that there was no difference in the protein level of GmGA2ox-like between WT and Gmilpa1-2 under white light (Fig. 4 i, k). However, GmGA2ox-like showed substantial degradation in WT exposed to white light supplemented with UV-B from 10 h, but not in Gmilpa1-2 under the same conditions (Fig. 4 i, l). In addition, we performed cell-free degradation assays using total protein extracts from WT or Gmilpa1-2 plants exposed to UV-B or maintained under white light and examined GmGA2ox-like abundance with anti-GmGA2ox-like. We did not observe degradation of GmGA2ox-like in either WT or Gmilpa1-2 extracts in the absence of UV-B (Supplementary Fig. 9b , d). However, GmGA2ox-like showed substantial degradation in WT extracts exposed to UV-B from 60 min, (Supplementary Fig. 9c , e), but not in Gmilpa1-2 extracts under the same conditions (Supplementary Fig. 9c , e). Incubation of MG132, an inhibitor of the 26 S proteasome degradation system, largely inhibited GmGA2ox-like degradation (Supplementary Fig. 9e ). We concluded that GmILPA1 promotes GmGA2ox-like degradation by a 26 S proteasome in UV-B-dependent manner. In light of the interaction of GmUBL1 with both GmILPA1 and GmGA2ox-like, we asked whether GmUBL1 played a role in GmGA2ox-like degradation with cell-free degradation assays using total protein extracts from N. benthamiana leaves transiently expressing GmUBL1 or GmGA2ox-like . We determined that GmUBL1 can’t promote the degradation of GmGA2ox-like directly, but requires GmILPA1 for this process (Fig. 4 j, m). The result showed that the protein degradation is apparent from 90 min to 150 min, and these results indicated that GmUBL1 enhanced the GmILPA1-mediated degradation of GmGA2ox-like. Gmilpa1-2 is sensitive to gibberellin and UV-B irradiation The phytohormone GA contributes to internode elongation. We thus treated H12 and Gmilpa1-2 soybean seedlings with 100 µmol GA 3 at the V1 stage (one unrolled trifoliate leaf) and measured plant height at the V4 stage (four unrolled trifoliate leaves). The results showed that exogenous GA 3 treatment restored Gmilpa1-2 height to that of H12 when grown under sunlight (Fig. 5a, b ). Treatment with the GA biosynthesis inhibitor paclobutrazol (PAC) efficiently inhibited elongation of H12, Gmilpa1-2 , and Gmilpa1 (Fig. 5c, d ). Additionally, the exogenous application of GA 3 rescued the PAC-induced growth deficiency of H12, Gmilpa1-2 , and Gmilpa1 seedlings and restored the dwarf phenotype of Gmilpa1-2 and Gmilpa1 treated with UV-B (Fig. 5c, d ). Fig. 5: Exogenous gibberellin application can rescue the dwarf phenotype of Gmilpa1-2 . a Phenotypes of Hedou 12 (H12) and Gmilpa1-2 seedlings grown under sunlight treated with GA 3 at the V1 stage (one unrolled trifoliate leaf), Scale bar, 20 cm. b Plant height of the seedlings at the V4 stage (three unrolled trifoliate leaves) in ( a ), ( n = 10 biologically independent samples; P = 1.92 × 10 −14 under mock condition). c Phenotypes of H12, Gmilpa1-2 , and Gmilpa1 seedlings treated with PAC alone and PAC with GA 3 treated with UV-B for 14 days, scale bar, 10 cm. d Plant height of the seedlings in ( c ), (n = 7 biologically independent samples; P = 1.12 × 10 −5 under UV-B condition). e – j Endogenous GA s levels in H12 and Gmilpa1-2 . 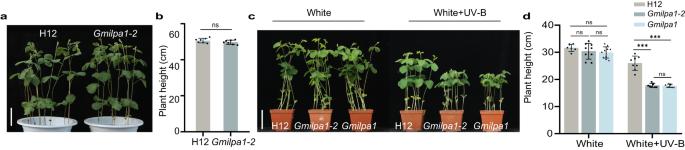Fig. 2: UV-B is required for theGmilpa1-2phenotype. aRepresentative image of the WT Hedou 12 (H12) andGmilpa1-2grown in a glasshouse at the V4 stage (four unrolled trifoliate leaves). Scale bar, 10 cm.bHeight of the plants shown in (a), (n= 7 biologically independent samples;P= 0.1909),P-values were calculated by comparing to H12 plants using two-tailed Student’st-test; ns not significant.cRepresentative images of the V2 stage of H12,Gmilpa1-2, andGmilpa1grown under white light (600 μmol m–2s–1white light, no UV-B, 25 °C, and a 12-h-light/12-h-dark photoperiod) and white light supplemented with UV-B (600 μmol m–2s–1white light, 1.5 μmol m−2s−1UV-B, 25 °C, and a 12-h-light/12-h-dark photoperiod). Scale bar, 10 cm.dHeight of the seedlings shown in (c), (n> 6 biologically independent samples;P= 2.42 × 10−6in H12 andGmilpa1-2,P= 1.80 × 10−6in H12 andGmilpa1). Data are presented as mean values ± SD;P-value is calculated with a one-way ANOVA analysis–Tukey comparison, and the columns labeled without the same alphabet are significantly different (P< 0.05, two-sided). ***P< 0.001, ns not significant. Source data are provided as a Source Data file. GA levels were measured using apical buds of V2-stage (two unrolled trifoliate leaves) seedlings grown under white light and white light with UV-B, ( n ≥ 3 biologically independent samples; P = 6 × 10 −4 in e P = 0.0134 in f P = 6.90 × 10 −6 in g P = 3.71 × 10 −7 in h P = 1.29 × 10 −7 in i P = 4 × 10 −4 in i ). P- values were calculated compared to H12 seedlings by two-tailed Student’s t -tests; *** P < 0.001, * P < 0.05; ns not significant. k Immunoblots showing GmILPA1 abundance in seedlings of H12 at the V1 stage (unrolled one trifoliate leaf) treated with 100 μM GA 3 and UV-B for the indicated times. l Phenotypes of H12, Gmilpa1-2 , and T 2 progeny lines of Gmilpa1-2/GmGA2ox-like RNAi grown under white light with UV-B (600 μmol m −2 s −1 , 1.5 μmol m −2 s −1 UV-B, 12-h light/12-h dark). Scale bar, 10 cm. m Plant height of the seedlings, ( n = 4 biologically independent samples for H12 and Gmilpa1-2 , n = 6 biologically independent samples for Gmilpa1-2/GmGA2ox-like-RNAi , P = 1.01 × 10 −4 in H12 and Gmilpa1-2 , P = 5.21 × 10 −4 in H12 and Gmilpa1-2/GmGA2ox-like-RNAi , P = 9.29 × 10 −5 in Gmilpa1-2 and Gmilpa1-2/GmGA2ox-like-RNAi ). In b , d , m , Data are presented as mean values ± SD, P- value is calculated with a one-way ANOVA analysis–Tukey comparison, and the columns labeled without the same alphabet are significantly different ( P < 0.05, two-sided). *** P < 0.001, ns, not significant. Source data are provided as a Source Data file. Full size image In addition, we measured the contents of endogenous GAs in H12 and Gmilpa1-2 under white light and white light supplemented with UV-B, such as bioactive GA 1 and GA 4 , as well as their precursors (GA 20 and GA 9 ) and catabolites (GA 8 and GA 34 ). In general, the endogenous GA content in both H12 and Gmilpa1-2 plants showed a decreasing trend under white light supplemented with UV-B (Fig. 5e–j ), which demonstrated that UV-B reduced the GA level in soybean. In addition, in consistent with the phenotype observed (Fig. 2c ), there was no difference in the levels of GAs between H12 and Gmilpa1-2 under white light, while the gibberellin GA 1 , GA 4 , GA 20 and GA 9 were more abundant in the WT plants than in Gmilpa1-2 under white light supplemented with UV-B conditions, the non-bioactive GA 8 and GA 34 accumulated at a relatively high level in Gmilpa1-2 relative to the H12 under same conditions (Fig. 5e–j ), indicating the reduction rate of active GA in Gmilpa1-2 was higher than that in H12. Therefore, our results demonstrated that GmILPA1 repressed the UV-B-induced decreasing of active GA levels to improve the UV-B tolerance in soybean. RT-qPCR analysis of GmILPA1 transcript levels in H12 seedlings treated with 100 µmol GA 3 and UV-B for 2, 4, 8, or 12 h indicated that GmILPA1 was significantly upregulated compared to the control after GA 3 treatment (Supplementary Fig. 10a ). However, relative GmILPA1 transcript levels did not respond to UV-B treatment in H12 (Supplementary Fig. 10b ). In addition, we observed that GmILPA1 accumulated within 12 h of treatment with GA 3 or UV-B light (Fig. 5m ). The results showed that GA 3 and UV-B induced GmILPA1 protein accumulation. In addition, RNA interference (RNAi) was used to silence GmGA2ox-like in Gmilpa1-2 , which was designated as Gmilpa1-2 / GmGA2ox-like RNAi . We grew H12, Gmilpa1-2 and Gmilpa1-2 / GmGA2ox-like RNAi seedlings under white light supplemented with UV-B, and the plant height of the T 2 generation of Gmilpa1-2 / GmGA2ox-like RNAi seedlings were significantly higher than that of Gmilpa1-2 (Fig. 5n, o , Supplementary Fig. 10c ), indicating that Gmilpa1-2 / GmGA2ox-like RNAi notably rescued the Gmilpa1-2 phenotype. Haplotypes 1, 2, 5 and 6 of GmILPA1 were selected during domestication and modern breeding efforts To understand the evolution of GmILPA1 during domestication, we investigated the selection signals over the promoter and genomic regions of GmILPA1 based on pairwise analyses of fixation index (FST), nucleotide diversity (π), and Tajima’s D values among 444 individuals wild, landrace, and improved cultivars (Fig. 6a , Supplementary Fig. 11a, b ). All three values across a 100-kb region containing GmILPA1 revealed a clear selective sweep from the promoter and genomic regions of GmILPA1 (Fig. 6a ). This result indicated that GmILPA1 underwent an artificial selection during soybean subsequent genetic improvement. To investigate the natural variation at GmILPA1 in germplasm resources, we performed a haplotype analysis across wild, landrace, and improved soybean populations [55] . We detected six main haplotypes, among which Hap5 (76.5%) and Hap1 (47.8%) mainly occurred in cultivated soybean, Hap2 (60.5%) and Hap6 (54.76%) were mainly present in landraces, and Hap3 and Hap4 were wild soybean-specific haplotypes (Fig. 6b ). To explore the evolution and spread of the six GmILPA1 haplotypes during soybean domestication and breeding, we constructed its corresponding phylogenetic tree and haplotype network using 444 accessions. The analysis indicated that Hap1–4 have a close genetic relationship, with Hap3 perhaps representing the ancestral alleles from which all other haplotypes derived, and Hap5 and Hap6 are closely related to the wild soybean-specific haplotypes Hap3 and Hap4 , respectively (Fig. 6c, d ). Fig. 6: Haplotype analysis and origin of GmILPA1 in soybean accessions from different populations of China. a FST, nucleotide diversity, and Tajima’s D values over the genomic region containing the GmILPA1 locus (~100 kb) between wild and cultivar soybean germplasms. b GmILPA1 haplotypes in natural populations. Top, schematic diagram of the GmILPA1 gene structure; gray, untranslated regions (UTRs); black, exons; black lines, promoter and introns. The CRE in the promoter region represents a light-responsive cis -regulatory element; –, 13-bp deletion. Bottom, GmILPA1 polymorphism across accessions relative to the Williams 82 reference genome ( Hap1 ). The number of varieties for each haplotype ( Hap1–6 ) is shown to the right. The cultivated soybean Hedou 12 belongs to Hap5 . c Evolutionary relationship of the GmILPA1 six haplotypes. d Haplotype origins of GmILPA1 as shown by the median-joining method. Circle size is proportional to the number of accessions, while circle colors represent the different soybean groups: blue, wild soybean ( S. soja ); green, landraces; magenta, cultivars. e – g Pie charts representing the distribution of each haplotype in wild soybeans, landraces, and improved cultivars. Full size image We also noticed that the number of haplotypes decreased from six in wild soybeans to four in the landraces and improved cultivars (Fig. 6e–g ), with the proportion of Hap1 Hap2 , Hap5 and Hap6 increasing from wild soybeans to the landraces, the proportion of Hap1 and Hap5 gradually increasing from wild soybeans to the landraces and to improved cultivars. The relative increase in Hap5 frequency was more substantial than the other haplotypes (Fig. 6e–g ), suggesting that mainly Hap1 and Hap5 , especially Hap5 , have been strongly selected for by humans during soybean domestication and modern breeding efforts. An INDEL in the GmILPA1 promoter confers variation of plant height in response to UV-B in cultivars Sequence analysis using the Plant-CARE database identified six Haps . Of them, Hap5 was the only haplotype with an INDEL (deletion of 13 bp) at position 1,877,295 bp (Indel-665) of the GmILPA1 promoter, which contains a light-responsive cis -regulatory elements (CREs). The deletion of this CRE may affect the transcriptional activity of GmILPA1 under UV-B conditions. We wished to investigate GmILPA1 transcriptional activity under UV-B stress. Accordingly, we cloned GmILPA1 promoters from Hap1 to Hap6 , and constructed their vectors GmILPA1pro Hap1 :GUS to GmILPA1pro Hap6 :GUS , and the GmILPA1 Hap5 promoter with indel vector GmILPA1pro Hap5/indel :GUS . We transiently expressed each construct in N. benthamiana leaves via Agrobacterium -mediated infiltration to test their transcriptional output with and without UV-B treatment. Histochemical staining showed no difference in GUS signal among GmILPA1pro Hap1 :GUS , GmILPA1pro Hap3 :GUS , GmILPA1pro Hap5 :GUS , GmILPA1pro Hap5/indel :GUS and GmILPA1pro Hap6 :GUS when infiltrated leaves were maintained under white light (Fig. 7a ). We also did not observe a difference in GUS signal for GmILPA1pro Hap5 :GUS regardless of UV-B exposure (Fig. 7a ). However, the GUS signal for GmILPA1pro Hap1 :GUS , GmILPA1pro Hap3 :GUS , GmILPA1pro Hap5/indel :GUS and GmILPA1pro Hap6 :GUS appeared higher than that of GmILPA1pro Hap5 :GUS when the infiltrated leaves were exposed to UV-B (Fig. 7a ). We confirmed these results with a quantitative GUS assay (Fig. 7b ). We performed RT-qPCR on the gene bar on the GUS vector as infiltration controls (Supplementary Fig. 12a ). These results suggested that the differential transcriptional activities between Hap5 and other haplotypes under UV-B expose is caused by the deletion of CRE in the GmILPA1 promoter of Hap5 , which has a significant effect on the response to UV-B. Fig. 7: Different Haplotypes of GmILPA1 confers variation of plant height in response to UV-B in cultivars. a GUS activity detected by histochemical staining in Nicotiana benthamiana leaves transiently expressing the GUS reporter gene under the control of GmILPA1 Hap1 - GmILPA1 Hap6 and the GmILPA1 Hap5 promoter with indel. For UV-B treatment, N. benthamiana were treated with UV-B (1.5 μmol m −2 s −1 ) for 12 h before histochemical staining. b GUS activity from N. benthamiana leaves transiently expressing GUS under the control of GmILPA1 Hap1 - GmILPA1 Hap6 and the GmILPA1 Hap5 promoter, as measured by fluorometric assay and expressed as pmol 4-methylumbelliferone μg –1 protein min –1 , ( n = 3 independent experiments, P = 0.0457 in Pro Hap1/2 : GUS, P = 0.0425 in Pro Hap3/4 : GUS, P = 0.0413 in Pro Hap6 : GUS and P = 0.0263 in Pro Hap5/indel : GUS). Data are presented as mean values ± SD, Student’s t -test was used for the significance test, ns, not significant, * P < 0.05. c–f Summary of major agronomic traits plants with the GmILPA1 Hap1 , GmILPA1 Hap2 , GmILPA1 Hap5 or GmILPA1 Hap6 allele. ( P = 0.0409 in Hap 1 and Hap 5, P = 0.0088 in Hap 6 and Hap 5, P = 0.0006 in Hap 2 and Hap 5) ( c ), ( P = 0.0233 in Hap 1 and Hap 5, P = 0.0017 in Hap 2 and Hap 5) ( d ), ( P = 2.61 × 10 −6 in Hap 1 and Hap 5, P = 3.57 × 10 −6 in Hap 6 and Hap 5, P = 8.95 × 10 −21 in Hap 2 and Hap 5) ( e ), ( P = 0.0143 in Hap 1 and Hap 5, P = 5.35 × 10 −6 in Hap 6 and Hap 5, P = 1.33 × 10 −6 in Hap 2 and Hap 5) ( f ). n = 179 for GmILPA1 Hap1 , n = 33 for GmILPA1 Hap2 , n = 76 for GmILPA1 Hap5 , n = 81 for GmILPA1 Hap6 . The box indicates the range from lower to upper quartiles, and the bar ranges the minimum to maximum observations; the significance of the difference is calculated by comparison with Hap 5 with a one-way ANOVA analysis–Tukey comparison and the columns labeled without the same alphabet are significantly different (P < 0.05, two-sided). * P < 0.05, ** P < 0.01, *** P < 0.001; ns, not significant. Source data are provided as a Source Data file. Full size image Modern breeding programs can progressively accumulate elite alleles. To further clarify whether accessions with improved cultivars differ from each other when grown under natural conditions, we measured their height. Haplotypes harboring Hap1 , Hap2 and Hap6 were taller than those with Hap5 (Fig. 7c ). We also investigated other agronomic traits in accessions carrying different haplotypes, which revealed that Hap5 generally have fewer pods, while hundred-seed weight and grain weight per plant were significantly higher than in other haplotypes (Fig. 7d–f ). These results suggested the high yield potential of Hap5 for soybean breeding programs. UV-B irradiation is an environmental stress that can inhibit the elongation of hypocotyls and stems, resulting in dwarf plants [56] . The regulation of hypocotyl elongation in response to UV-B light is usually mediated by its dedicated photoreceptor UVR8 [32] , [33] , [35] , [57] and the E3 ligase CONSTITUTIVELY PHOTOMORPHOGENIC1 (COP1), which binds to UVR8 monomers to initiate UV-B signaling [57] , [58] . However, whether other E3 ligases are involved in plant height in response to UV-B is unknown. In this study, we identified a subunit of the APC/C in soybean, GmILPA1, as an APC8-like protein with E3 ubiquitin ligase activity. We also showed that UV-B can promote the accumulation of GmILPA1 to control plant height of soybean under UV-B exposure (Figs. 2a, c and 5k ). Thus, GmILPA1 might be involved in UV-B acclimation in soybean. So far, little is known about plant targets of the APC/C compared to their counterparts in animals and yeast ( Saccharomyces cerevisiae ). Known substrates of the APC/C in plants include cyclin (CYCA3;1/CYCA2;3) and CYCB2;1 [59] , [60] , [61] , the double-stranded (ds) RNA-Binding Protein 4 (DRB4) [62] , a member of the plant-specific GRAS family MONOCULM1 (MOC1) [63] , and a small GTP binding protein ROOT ARCHITECTURE-ASSOCIATED1 (RAA1) [64] , [65] , [66] . In this study, we identified GmGA2ox-like as an interacting protein of GmILPA1 in a yeast two-hybrid screen (Fig. 3a ). GmGA2ox-like harbors the typical D-box (the destruction box, RXXLXXXN) that is recognized and degraded by the APC/C (Supplementary Fig. 6f ). Further we found that GmGA2ox-like was recognized by GmILPA1 (APC/C) and degraded only upon UV-B exposure in soybean (Fig. 4i ). Therefore, we indicated that GmGA2ox-like is a novel substrate of the APC/C. A previous study showed that UV-B-induced morphological adjustments are associated with the dynamic stability in phytohormones like GA [37] . UV-B induces the expression of the GA catabolic genes GA2ox2 and GA2ox8 in Arabidopsis , thus inhibiting hypocotyl elongation, and UV-B influences the expression of GA metabolic genes requiring UVR8 [67] , [68] . However, whether GA2ox function is also modulated at the post-transcriptional level has remained unclear. In this study, we found that GmGA2ox-like is recognized by the APC/C and degraded only upon UV-B exposure in soybean (Fig. 4i ), and indicated that the degradation of GmGA2ox-like by GmILPA1 is UV-B dependent. Moreover, we found that another E3 ligase GmUBL1 also interacted with GmGA2ox-like and ubiquitinated GmGA2ox-like, which further promoted the degradation of GmGA2ox-like (Fig. 4j ). We speculated that the enhanced ubiquitination of GmGA2ox-like further accelerates its degradation. Furthermore, the levels of active GAs in the Gmilpa1-2 mutant were significantly lower than in the WT (Fig. 5e, f ), and exogenous GA applications restored the height of the Gmilpa1-2 mutant to that of the WT under UV-B light (Fig. 5c ). In agreement with these results, overexpression of GmGA2ox-like led to dwarfism in soybean (Supplementary Fig. 6d ), similar to the Gmilpa1-2 mutant. By measuring the GAs contents in WT and Gmilpa1-2 plants, we found that UV-B-induced reduction rate of active GA in Gmilpa1-2 was higher than that in H12 (Fig. 5e–j ). Therefore, we demonstrated that GmILPA1-GmGA2ox-like module enhances the UV-B tolerance to maintain growth in soybean by repressing UV-B-induced reduction of active GA levels. Taken together, these findings improve our understanding of the mechanisms that how soybean plants improve its tolerance to UV-B stress. Interestingly, exogenous GA only restored the plant height of Gmilpa1-2 , while Gmilpa1-2 plants was different with wild type for the overall morphology (Fig. 5a ). Considering the importance of hormone homeostasis, we hypothesize that this phenomenon might be GA-dose dependent. Moreover, previous study reported that GA treatment did not restore the petiole angle of the Gmssp ( Gmilpa1 ) mutant [69] . 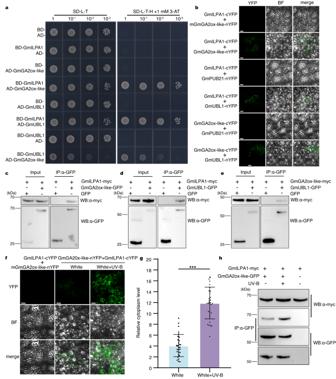Fig. 3: GmILPA1 interacts with GmGA2ox-like and GmUBL1. aYeast two-hybrid assays showing the interactions among GmILPA1, GmGA2ox-like, and GmUBL1. GmILPA1 and GmUBL1 were fused to GAL4-BD, and GmGA2ox-like was fused to GAL4-AD when encoded by the pGADT7 and pGBKT7 vectors. Serial dilutions of equivalent amounts of yeast were plated on synthetic defined (SD) medium without Leu (L), Trp (T) (SD-L-T), or without Leu (L), Trp (T), and His (H) (SD-L-T-H) containing 1 mM 3-amino-1,2,4-triazole (3-AT), with growth on triple dropout media indicating an interaction between the tested proteins.bA BiFC assay used to verify the interactions among GmILPA1, GmGA2ox-like, and GmUBL1 in vivo inN. benthamianaleaves. The non-interacting proteins, mGmGA2ox-like (mutated construct of D-Box motif) and GmPUB21 (a U-Box E3 Ubiquitin Ligases), were used as a negative control. Scale bars, 50 μm.c–eCo-IP of GmILPA1, GmGA2ox-like, and GmUBL1. Immunoprecipitation was performed with anti-GFP-agarose beads usingN. benthamianaleaves co-infiltrated with the constructsGmGA2ox-like-GFPandGmILPA1-MYC(c),GmUBL1-GFPandGmILPA1-MYC(d), orGmUBL1-GFPandGmGA2ox-like-MYC(e).fBiFC assays indicating that UV-B treatment promotes the interaction between GmILPA1 and GmGA2ox-like.N. benthamianaleaves were co-infiltrated withGmGA2ox-like–nYFPandGmILPA1–cYFPand exposed to 1 h of UV-B (21 μmol m−2s−1) or kept in white light before imaging. Scale bars, 50 μm.gRelative YFP fluorescence intensity in the cytoplasm from the images in (f), (n= 30 cells,P= 1.30 × 10−5), the relative fluorescence intensities of cytoplasm and whole cells were quantified and the cytoplasm-to- background ratios are plotted. Data are presented as mean values ± SD, Student’st-test was used for the significance test, ***P< 0.001.hCo-IP assays showed that UV-B increased the interaction between GmILPA1 and GmGA2ox-like.N. benthamianawere co-transformed withGmGA2ox-like-GFPandGmILPA1-MYC, and treated with or without 12 h UV-B. Then, they were used in the co-immunoprecipitation assay. Immunoprecipitation was performed using GFP-Trap agarose beads, and the immunoblots were probed using anti-myc and anti-GFP antibodies. Source data are provided as a Source Data file. Therefore, in addition to mediating plant height via GA metabolism, GmILPA1 might be involved in different growth and development processes, such as leaf petiole angle regulation, through other mechanisms. Although E3 ligase itself has ubiquitination ligase activity and is able to ubiquitinate substrates, it may also be regulated by other proteins. For example, SPA can interact with COP1 and enhance the ubiquitination activity of COP1 in vitro [70] , while COP1 can be ubiquitinated and degraded mediated by CSU1 (a RING-finger E3 ubiquitin ligase) in darkness [71] . In this study, we identified another E3 ligase GmUBL1 as an interacting protein of GmILPA1 and GmGA2ox-like (Fig. 3a ). GmUBL1 could induce the ubiquitination of GmGA2ox-like but did not lead to degradation of GmGA2ox-like (Fig. 4j ). Further studies demonstrated that GmUBL1 promoted the GmILPA1-mediated degradation of GmGA2ox-like, probably due to enhanced ubiquitination (Fig. 4j ). Therefore, we speculate that GmUBL1 might enhance the ubiquitin E3 ligase activity of GmILPA1, suggesting a more complicated regulation mechanism for GmILPA1 activity and GmGA2ox-like stability. Achieving ideal plant architecture is an important objective of artificial selection and modern breeding, as it can increase grain yield by allowing denser planting and raising photosynthetic efficiency [72] . Due to artificial selection of specific alleles (haplotypes) during crop domestication and breeding, plants with new traits meeting human needs were produced, but this is often accompanied by a loss of allele diversity [73] . In this study, we detected evidence of artificial selection over the GmILPA1 locus during soybean domestication and modern genetic improvement. We showed that Hap1 and Hap5 were the main selected haplotypes in modern cultivated germplasms, while Hap2 and Hap6 gradually declined in frequency from wild soybeans to modern cultivated germplasms (Fig. 6c–e ). This pattern suggested that Hap1 and Hap5 are haplotypes that have mainly undergone artificial selection. Mutations in exons that lead to loss of function often cause strong phenotypic changes, but alterations in transcription levels are also an important genetic basis for trait transition [74] . The selection of Hap5 in modern improved cultivars may be associated with the light-responsive CRE present in Hap1 , Hap2 and Hap6 , but not in Hap5 ; notably, relative GmILPA1 transcript activity was higher harboring Hap1 , Hap2 , and Hap6 compared with those with Hap5 upon exposure to UV-B in the N. benthamiana transient expression system (Fig. 7a, b ), indicating that the deletion of the light-responsive cis -regulatory element CRE may affect the response to UV-B. Further we also investigated plant height in accessions carrying different haplotypes, and found that Hap5 with the deletion of CRE generally is shorter than other haplotypes (Fig. 7a ). Together, these results suggested the INDEL in the GmILPA1 promoter may be involved in this phenotypic difference. Given that northern China has more ultraviolet radiation than southern China [75] , we surveyed the geographical distribution of Hap1 , Hap5 and Hap6 using soybean cultivars collected from 7 geographical regions in northern China (Jilin, Liaoning and Heilongjiang provinces) and southern China (Fujian, Guizhou, Jiangxi and Hunan provinces). The frequency of Hap1 and Hap6 increased from the north region to the south region. By contrast, Hap5 only appears in the north of China (Fig. 8a ), suggesting that the growth of Hap5 is more suitable for high UV-B environments. Furthermore, we analyzed GmILPA1 transcript levels after UV-B treatment in 30 randomly selected soybean accessions each for Hap1 and Hap5 . We observed that GmILPA1 from Hap1 germplasm is more highly expressed than in Hap5 germplasm in response to UV-B light (Supplementary Fig. 12b ). In addition, we measured plant height for all 60 accessions grown under white light only or exposed to UV-B light. Notably, plant height for Hap1 germplasms was significantly higher than that of Hap5 germplasms upon exposure to UV-B light (Supplementary Fig. 12c ). Therefore, we speculated that the deletion of CRE in GmILPA1 promoter of Hap5 leads to the reduction of plant height under UV-B radiation, which is a manifestation of the soybean’s own protection resistant to UV-B radiation (Fig. 8b ). Taken together, Hap5 variant could be used to develop new soybean cultivars with ideotype and tolerant to UV-B radiation. Importantly, GmILPA1 is held to be a promising potential target for single base editing aimed at raising the planting density and lodging-resistant of soybean in the future. Fig. 8: A working model of the regulation of plant height by the GmILPA1-GmUBL1-GmGA2ox-like module in soybean. a Geographical distribution of Hap1 , Hap5 and Hap6 . N, north of China, S, south of China. The pie chart represents their frequency. b The working model of GmILPA1 regulating of plant height in Hap1 / 2 / 6 and Hap5 . In Hap1 / 2 / 6 , under the UV-B irradiation, GmILPA1 accumulation is induced at transcriptional and protein levels. GmGA2ox-like is ubiquitinated by GmILPA1 and GmUBL1, and GmILPA1 mediates the degradation of GmGA2ox-like, GmUBL1 enhanced the degradation of GmGA2ox-like. As a result, the increase of bioactive GAs content promoted the growth of soybean. In Hap5 , under the UV-B irradiation, GmILPA1 accumulation is induced only at protein level, eventually leads to shorter plant height in Hap5 . GA3 induces GmILPA1 protein accumulation both in Hap1 / 2 / 6 and Hap5 . Full size image Plant materials and growth conditions The Gmuid1 (also named Gmilpa1-2 ) mutant was generated in our laboratory; Gmilpa1 was provided by Xianzhong Feng. Both mutants are in the soybean ( Glycine max L.) Heidou 12 background. To investigate the phenotype of Hedou 12 and Gmuid1 under natural sunlight (70–100 μW cm –2 UV-B), plants were grown at Qingdao, Shandong (35.35° N, 119.3° E) during the summer. The UV intensity was measured using a 254 UV light meter (manufactured by Beijing Normal University). For laboratory experiments, plants were cultivated in a glasshouse (with no UV-B) under natural sunlight and in a phytotron equipped with LED lights. For treatments with white light, Hedou 12 and the Gmuid1 mutant were grown in a growth chamber (600 μmol m –2 s –1 white light, no UV-B, 25 °C, 12-h-light/12-h-dark photoperiod). For UV-B treatment, weak narrow-band UV-B coupled with white light was used (600 μmol m –2 s –1 white light, 1.5 μmol m −2 s −1 ; TL20W/01RS tubes, Philips; 12-h-light/12-h-dark photoperiod). For treatment with gibberellin, the leaves of V1-stage plants were sprayed with 100 μM GA 3 (Sigma-Aldrich, USA) using a hand-held aerosol-propelled sprayer, spray plants with water as negative control Map-based cloning of GmILPA1 ( GmUID1 ) For map-based cloning of GmILPA1 , an F 2 population was generated by crossing the Gmuid1 mutant in the Heidou 12 background and Williams 82. F2 plants with the mutant phenotype were used for mapping with the markers listed in Supplementary Data 2 . For bulk segregant analysis, 80 plants (40 with a wild-type phenotype and 40 with the mutant phenotype) were selected from the F 2 population. Genomic DNA was extracted from all individual plants and mixed in equal amounts to generate the wild-type pool (W-pool) and the mutant pool (M-pool). Sequencing libraries were constructed for each pool and the parents Heidou 12 and Williams 82. Genomic DNA was sheared for preparation of the sequencing library according to the standard protocol of the Illumina TruSeq DNA PCR-free prep kit. Reads of the two bulks and the parental line were aligned to the reference genome using bwa software with default parameters; SNP calling was performed using GATK software. SNPs with a sequencing depth of <5 were filtered. Then, the SNP index was calculated, and SNPs with a SNP index of <0.3 in both bulks were filtered to reduced false positive detection of SNPs. Statistical confidence intervals of Δ (SNP index) were calculated under the null hypothesis of no quantitative trait loci (QTLs) following procedures reported previously [76] . The primers are listed in Supplementary Data 2 . Plasmid construction and transformation The coding sequences of GmILPA1 and GmGA2ox-like were amplified from Hedou 12 complementary DNA (cDNA) and cloned in-frame with the GFP coding sequence into the pB7FWG2 vector under the control of the cauliflower mosaic virus (CaMV) 35S promoter. The resulting constructs were introduced into the Gmilpa1-2 mutants and Hedou 12 by Agrobacterium ( A. tumefaciens )–mediated transformation. The primers are listed in Supplementary Data 2 . RNA extraction and RT-qPCR Total RNA from examined organs was isolated using Trizol reagent (Invitrogen). First-strand cDNA was synthesized from 1 µg of total RNA using a MonScript RTIII All-in-One Mix with dsDNase (Monad). For qPCR, each sample was subjected to three technical replicates, using a 2× M5 HiPer Realtime PCR Super Mix on an Applied Biosystems instrument. The level of GmELF1b was used as the internal control [77] . GA measurements To quantify the contents of GAs, H12 and Gmilpa1-2 seedlings were grown under white light and white light with UV-B. The stem apexes of the seedlings were collected, frozen in liquid nitrogen, ground to a fine powder, and extracted with the traction method (methanol/water/formic acid = 15:4:1, V/V/V). The extracts were vortexed and centrifuged at 4694 × g under 4 °C for 10 min. The supernatants were dried by evaporation under the flow of nitrogen gas at room temperature, then dissolved in 200 μl of methanol. The sample extracts were analyzed using an LC-ESI-MS/MS system (HPLC, Shimpack UFLC SHIMADZU CBM30A system; MS, Applied Biosystems 6500 Triple), and the data were analyzed by Metware Biotechnology Co., Ltd (Wuhan, China). At least three replicates of each assay were performed, the information of ions monitored was provided in Supplementary Data 1 . Immunoblotting Total proteins were extracted with extraction buffer (50 mM Tris-HCl, pH 7.5, 150 mM NaCl, 5 mM EDTA, 2 mM DTT, 10% [v/v] glycerol, 1 mM PMSF, 1% [v/v] PVPP, and 1× protease inhibitor cocktail). Samples were immediately boiled for 10 min and then centrifuged at 14,000 × g for 10 min at room temperature. Proteins from the supernatant were used for immunoblotting. The anti-GmILPA1 and anti-GmGA2ox-like antibodies were produced by MW BIOTECH (HK) LIMITED. Yeast two-hybrid and bimolecular fluorescence complementation (BiFC) assays The full-length coding sequences of GmILPA1 , GmGA2ox-like , and GmUBL1 were cloned into pGADT7 or pGBKT7 vectors to generate the bait and prey constructs, respectively. The appropriate pairs of constructs were co-transformed into yeast strain Y2HGold and grown on selective plates at 30 °C for 2–4 days. For BiFC assays, the same coding sequences were cloned in-frame with the nYFP or cYFP sequences to generate GmILPA1-cYFP , GmGA2ox-like-nYFP , GmGA2ox-like-cYFP , and GmUBL1-nYFP . The resulting constructs were transformed into Agrobacterium strain GV3101, and the appropriate pairs were co-infiltrated into N. benthamiana leaves together with the silencing suppressor P19. 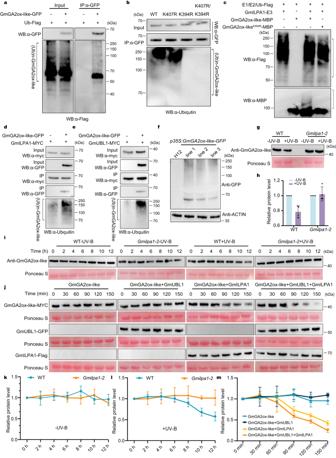Fig. 4: GmGA2ox-like is ubiquitinated and degraded by the proteasome. aIn vivo ubiquitination of GmGA2ox-like as detected by co-immunoprecipitation (Co-IP) assay.bIdentification of the ubiquitination sites essential for GmGA2ox-like ubiquitination.cUbiquitination of GmGA2ox-like by GmILPA1 in vitro. Brackets denote the ubiquitinated bands.d,eUbiquitination of GmGA2ox-like by GmILPA1 inN. benthamianaleaves viaAgrobacterium-mediated transient expression.fGmGA2ox-like is ubiquitinated in plants. Ubiquitinated proteins were enriched from the P62-agarose matrix that was incubated with total proteins isolated from three independent transgenic plants stably expressingGmGA2ox-like-GFPor from H12 plants.gRegulation of GmGA2ox-like stability byGmILPA1in vivo. H12 andGmilpa1-2seedlings grown under white light and white light supplemented with UV-B to the V2 stage, and GmGA2ox-like was checked with an anti-GmGA2ox-like antibody. The band intensities in western blots were quantified (h), Data are presented as mean values ± SEM,n= 3 independent experiments.iImmunoblots showing GmGA2ox-like protein levels in V2 stage seedlings of H12 andGmilpa1-2grown in white light (600 μmol m−2s−1, 12 h/12 h light/dark) and then transferred to white light supplemented with UV-B (1.5 μmol m−2s−1, 12 h/12 h light/dark) for the indicated time periods. GmGA2ox-like abundance was detected with anti-GmGA2ox-like antibody and quantified (k,l). Data are presented as mean values ± SEM,n= 3 independent experiments.jGmGA2ox-like degradation in cell-free degradation assays in the presence of GmILPA1 and GmUBL1.GmGA2ox-like-MYC,GmUBL1-GFP, andGmILPA1-FLAGwere individually infiltrated inN. benthamiana.GmGA2ox-like-MYCprotein extracts were individually mixed with recombinantGmUBL1-GFP,GmILPA1-FLAG, GmUBL1-GFP, orGmILPA1-FLAG. Samples were collected at the indicated time points, and GmGA2ox-like abundance was probed by immunoblotting with anti-MYC antibody and quantified (m). Data are presented as mean values ± SEM,n= 3 independent experiments. Source data are provided as a Source Data file. Fluorescent signals were visualized by using the LSM-700 laser scanning confocal microscope (Zeiss) and the signal intensities of YFP were determined by ImageJ software. The primers used in the generation of the relevant construct are listed in Supplementary Data 2 . Microscopy procedures To observe longitudinal parenchyma cells of H12 and Gmuid1 , the fifth internode was fixed in FAA solution (5% formaldehyde, 50% absolute alcohol, 5% acetic acid) and then embedded in paraffin using a HistoCore Arcadia machine (Leica Biosystems). Sections (7 μm in thickness) were obtained using a HistoCore MULTICUT (Leica Biosystems) and observed and photographed using a microscope (Olympus BX51) with a DP72 camera (Olympus). For the YFP fluorescence signals, fluorescence microscopy of abaxial leaf epidermal cells was performed using a confocal laser scanning microscope (ZEISS LSM 700; ZEISS, Oberkochen, Germany). Co-immunoprecipitation (Co-IP) assays The CDSs of GmGA2ox-like and GmUBL1-GFP were cloned into the modified vector to generate GmGA2ox-like-GFP and GmUBL1-GFP . The CDS of GmILPA1 and GmGA2ox-like were cloned into the modified vector to generate GmILPA11-myc and GmGA2ox-like-myc . 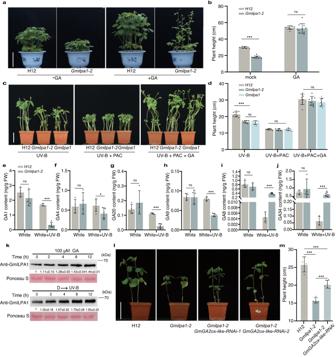Fig. 5: Exogenous gibberellin application can rescue the dwarf phenotype ofGmilpa1-2. aPhenotypes of Hedou 12 (H12) andGmilpa1-2seedlings grown under sunlight treated with GA3at the V1 stage (one unrolled trifoliate leaf), Scale bar, 20 cm.bPlant height of the seedlings at the V4 stage (three unrolled trifoliate leaves) in (a), (n= 10 biologically independent samples;P= 1.92 × 10−14under mock condition).cPhenotypes of H12,Gmilpa1-2, andGmilpa1seedlings treated with PAC alone and PAC with GA3treated with UV-B for 14 days, scale bar, 10 cm.dPlant height of the seedlings in (c), (n = 7 biologically independent samples;P= 1.12 × 10−5under UV-B condition).e–jEndogenous GAslevels in H12 andGmilpa1-2. GA levels were measured using apical buds of V2-stage (two unrolled trifoliate leaves) seedlings grown under white light and white light with UV-B, (n≥ 3 biologically independent samples;P= 6 × 10−4ineP= 0.0134 infP= 6.90 × 10−6ingP= 3.71 × 10−7inhP= 1.29 × 10−7iniP= 4 × 10−4ini).P-values were calculated compared to H12 seedlings by two-tailed Student’st-tests; ***P< 0.001, *P< 0.05; ns not significant.kImmunoblots showing GmILPA1 abundance in seedlings of H12 at the V1 stage (unrolled one trifoliate leaf) treated with 100 μM GA3and UV-B for the indicated times.lPhenotypes of H12,Gmilpa1-2, and T2progeny lines ofGmilpa1-2/GmGA2ox-like RNAigrown under white light with UV-B (600 μmol m−2s−1, 1.5 μmol m−2s−1UV-B, 12-h light/12-h dark). Scale bar, 10 cm.mPlant height of the seedlings, (n= 4 biologically independent samples for H12 andGmilpa1-2,n= 6 biologically independent samples forGmilpa1-2/GmGA2ox-like-RNAi,P= 1.01 × 10−4in H12 andGmilpa1-2,P= 5.21 × 10−4in H12 andGmilpa1-2/GmGA2ox-like-RNAi,P= 9.29 × 10−5inGmilpa1-2andGmilpa1-2/GmGA2ox-like-RNAi). Inb,d,m, Data are presented as mean values ± SD,P-value is calculated with a one-way ANOVA analysis–Tukey comparison, and the columns labeled without the same alphabet are significantly different (P< 0.05, two-sided). ***P< 0.001, ns, not significant. Source data are provided as a Source Data file. The GmILPA1-myc , GmGA2ox-like-GFP , GmUBL1-GFP , or GmGA2ox-like-myc construct was transformed into Agrobacterium strain GV3101. Agrobacteria harboring the indicated constructs were co-infiltrated into the epidermal cells of N. benthamiana leaves. 100 μM MG132 was co-injected with the Agrobacterium suspension to prevent the degradation of GmGA2ox-like-GFP protein. The plants were grown for 3 days at 25 °C before the infiltrated leaves were collected. Total proteins were extracted in extraction buffer containing 20 mM HEPES, pH 7.4, 150 mM NaCl, 1 mM EDTA, 0.5% (v/v) Triton X-100, 1 mM PMSF, 10% (v/v) glycerol, 1× protease inhibitor cocktail, and 0.1% (v/v) β-mercaptoethanol. After centrifugation for 15 min at 14,000 × g at 4 °C. The supernatant was mixed with 15 μl of anti-GFP-conjugated agarose beads (Chromotek), incubated at 4 °C for 3 h, and washed four times with washing buffer (20 mM HEPES, pH 7.4, 150 mM NaCl, 1 mM EDTA, 0.5% [v/v] Triton X-100, 1 mM PMSF, and 1×protease inhibitor cocktail). The bound proteins were eluted from the beads in 4× SDS-PAGE sample buffer and analyzed by immunoblot using anti-Myc (Proteintech, 60003-2-Ig, 1:5000(v/v)) or anti-GFP (Proteintech, 66002-1-Ig, 1:5000(v/v)) antibodies. The primers used in the generation of the relevant construct are listed in Supplementary Data 2 . In vitro ubiquitination assay The assay was performed as described previously with minor modifications [78] . Purified recombinant GmGA2ox-like-MBP (maltose binding protein) was used as substrate and GmILPA1-GFP as E3, GmILPA1 was immunopurified as the E3 from transgenic plants of 35S:GmILPA1-GFP using GFP-Trap agarose beads (Chromotek). The other ingredients, including E1, E2 (UbcH5b/UBE2D2), and ubiquitin (Ub), were purchased from Boston Biochem (Cambridge, MA). Ubiquitination assays were performed in reaction buffer containing 50 mM Tris-HCl, pH 7.5, 5 mM MgCl 2 , 2 mM ATP, 2 mM dithiothreitol (DTT), and 20 μM MG132. After 2 h of incubation at 30 °C, the reaction was stopped by adding SDS loading buffer. Ubiquitinated GmGA2ox-like-MBP was detected by immunoblotting with anti-Ub (Proteintech, 10201-2-AP, 1:1000(v/v)) and anti-MBP (Proteintech, 66003-1-Ig, 1:5000(v/v)) antibodies. Determinant amino acids of GmGA2ox-like responsible for the ubiquitination were identified using an online prediction website (gpsuber.biocuckoo.cn/). In vivo ubiquitination assay The assay was performed as described previously with minor modifications [79] . For the in vivo ubiquitination assay of GmGA2ox-like and GmILPA1, cultures of Agrobacterium strain GV3101 harboring the constructs GmGA2ox-like-GFP and Ub-flag , GmGA2ox-like and GmUBL1 , GmILPA1 and GmGA2ox-like-GFP , GmGA2ox-like-GFP , GmGA2ox-like K407R -GFP , GmGA2ox-like K394R -GFP , and GmGA2ox-like K394R,K407R -GFP were infiltrated into N. benthamiana leaves. 100 μM MG132 was co-injected with the Agrobacterium suspension to prevent the degradation of GmGA2ox-like-GFP protein. Leaf tissues were harvested 2 days after infiltration, and total proteins were extracted with extraction buffer (20 mM HEPES, pH 7.4, 150 mM NaCl, 1 mM EDTA, 0.5% [v/v] Triton X-100, 1 mM PMSF, 10% [v/v] glycerol, 1× protease inhibitor cocktail, and 0.1% [v/v] β-mercaptoethanol). The supernatant was mixed with 15 μl of anti-GFP-conjugated agarose beads (Chromotek) for 3 h at 4 °C. The beads were washed at least three times with washing buffer, followed by elution in 4× loading buffer and separation by SDS-PAGE and detection by immunoblotting using anti-FLAG (Proteintech, 66008-4-Ig, 1:1000(v/v)) or anti-ubiquitin antibodies (Proteintech, 10201-2-AP, 1:1000(v/v)). The primers used in the generation of the relevant constructs are listed in Supplementary Data 2 Cell-free degradation assay The assay was performed as described previously with minor modifications [80] . For the degradation of GmGA2ox-like in soybean, total proteins were extracted from Hedou 12 and Gmilpa1-2 leaves using extraction buffer (50 mM Tris-MES, pH 8.0, 0.5 mM sucrose, 1 mM MgCl 2 , 10 mM EDTA, and 5 mM DTT with freshly added protease inhibitor cocktail). After centrifugation for 15 min at 14,000 × g at 4 °C. The protein extracts were then incubated with 10 mM ATP at 25 °C for 0 to 90 min in the presence or absence of 50 μM MG132. The abundance of GmGA2ox-like was determined by immunoblotting. For the degradation of GmGA2ox-like in N. benthamiana , total proteins extracted from leaves infiltrated with GmILPA1-flag or GmUBL1-GFP or from the leaves of non-infiltrated (control) N. benthamiana leaves were mixed with total proteins extracted from N. benthamiana leaves expressing GmGA2ox-like-myc . A final concentration of 10 mM ATP was added to the cell lysates to preserve the function of the 26 S proteasome before incubation for the indicated times at 25 °C. GmGA2ox-like-myc, GmILPA1-flag, and GmUBL1-GFP protein levels were analyzed by immunoblotting with anti-GFP (Proteintech, 66002-1-Ig, 1:5000(v/v)), anti-Myc (Proteintech, 60003-2-Ig, 1:5000(v/v)), and anti-Flag (Proteintech, 66008-4-Ig, 1:1000(v/v)) antibodies, respectively. The primers used in the generation of the relevant construct are listed in Supplementary Data 2 . Affinity purification of ubiquitinated proteins Total proteins of Wild-type and three P35S:GmGA2ox-like-GFP transgenic plants were extracted with 1 ml of BI buffer (50 mM Tris-HCl, (pH 7.5), 20 mM NaCl, 0.1% NP-40 and 5 mM ATP) in a prechilled mortar. The following were added to the protein homogenates: 1 mM PMSF, 50 mM MG132, 10 nM Ub aldehyde, and 10mM N-ethylmaleimide. Protein extracts were incubated with 40 μL of prewashed p62-agarose (Enzo Life Sciences, cat. no. BML-UW9010-0500) in 2 ml of BI buffer at 4 °C. After 4 h, the agaroses were washed two times with BI buffer and once with BII buffer (supplemented with 200 mM NaCl in BI). Samples were boiled in 50 μL of 1×SDS loading buffer for 5 min. The ubiquitinated proteins were separated by 10% SDS–PAGE gel, and anti-GFP antibody was used to detect ubiquitinated GmGA2ox-like-GFP protein. 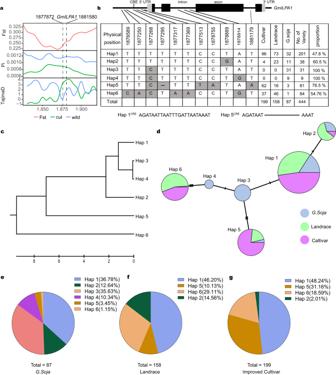Fig. 6: Haplotype analysis and origin ofGmILPA1in soybean accessions from different populations of China. aFST, nucleotide diversity, and Tajima’s D values over the genomic region containing theGmILPA1locus (~100 kb) between wild and cultivar soybean germplasms.bGmILPA1haplotypes in natural populations. Top, schematic diagram of theGmILPA1gene structure; gray, untranslated regions (UTRs); black, exons; black lines, promoter and introns. The CRE in the promoter region represents a light-responsivecis-regulatory element; –, 13-bp deletion. Bottom,GmILPA1polymorphism across accessions relative to the Williams 82 reference genome (Hap1). The number of varieties for each haplotype (Hap1–6) is shown to the right. The cultivated soybean Hedou 12 belongs toHap5.cEvolutionary relationship of theGmILPA1six haplotypes.dHaplotype origins ofGmILPA1as shown by the median-joining method. Circle size is proportional to the number of accessions, while circle colors represent the different soybean groups: blue, wild soybean (S. soja); green, landraces; magenta, cultivars.e–gPie charts representing the distribution of each haplotype in wild soybeans, landraces, and improved cultivars. Haplotype of GmILPA1 For the investigation of the natural variation at GmILPA1 , a panel of 444 soybean accessions consisting of 87 wild, 158 landrace, and 199 cultivated soybeans were subjected to haplotype analysis. A total of 10 SNPs and 1 InDel in the 5.7-kb region surrounding GmILPA1 were used for haplotype classification. Six main haplotypes were obtained based on qualified genotypic and phenotypic data for GmILPA1 . The remaining haplotypes were represented by fewer accessions, were deemed rare, and thus were not considered in this study. Haplotype network analysis was performed using PopART software based on the ‘Median-Joining Network’ approach. 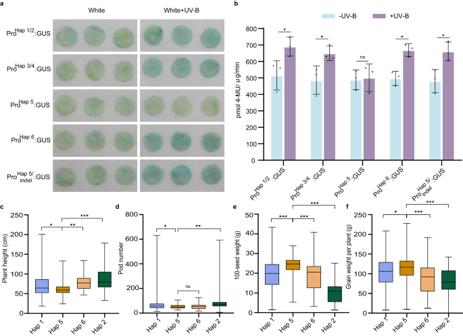Fig. 7: Different Haplotypes ofGmILPA1confers variation of plant height in response to UV-B in cultivars. aGUS activity detected by histochemical staining inNicotiana benthamianaleaves transiently expressing theGUSreporter gene under the control ofGmILPA1Hap1- GmILPA1Hap6and theGmILPA1Hap5promoter with indel. For UV-B treatment,N. benthamianawere treated with UV-B (1.5 μmol m−2s−1) for 12 h before histochemical staining.bGUS activity fromN. benthamianaleaves transiently expressingGUSunder the control ofGmILPA1Hap1- GmILPA1Hap6and theGmILPA1Hap5promoter, as measured by fluorometric assay and expressed as pmol 4-methylumbelliferone μg–1protein min–1, (n= 3 independent experiments,P= 0.0457 in ProHap1/2: GUS,P= 0.0425 in ProHap3/4: GUS,P= 0.0413 in ProHap6: GUS andP= 0.0263 in ProHap5/indel: GUS). Data are presented as mean values ± SD, Student’st-test was used for the significance test, ns, not significant, *P< 0.05.c–fSummary of major agronomic traits plants with theGmILPA1Hap1,GmILPA1Hap2, GmILPA1Hap5orGmILPA1Hap6allele. (P= 0.0409 in Hap 1 and Hap 5,P= 0.0088 in Hap 6 and Hap 5,P= 0.0006 in Hap 2 and Hap 5) (c), (P= 0.0233 in Hap 1 and Hap 5,P= 0.0017 in Hap 2 and Hap 5) (d), (P= 2.61 × 10−6in Hap 1 and Hap 5,P= 3.57 × 10−6in Hap 6 and Hap 5,P= 8.95 × 10−21in Hap 2 and Hap 5) (e), (P= 0.0143 in Hap 1 and Hap 5,P= 5.35 × 10−6in Hap 6 and Hap 5,P= 1.33 × 10−6in Hap 2 and Hap 5) (f).n= 179 forGmILPA1Hap1,n= 33 forGmILPA1Hap2,n= 76 forGmILPA1Hap5,n= 81 forGmILPA1Hap6. The box indicates the range from lower to upper quartiles, and the bar ranges the minimum to maximum observations; the significance of the difference is calculated by comparison with Hap 5 with a one-way ANOVA analysis–Tukey comparison and the columns labeled without the same alphabet are significantly different (P < 0.05, two-sided). *P< 0.05, **P< 0.01, ***P< 0.001; ns, not significant. Source data are provided as a Source Data file. 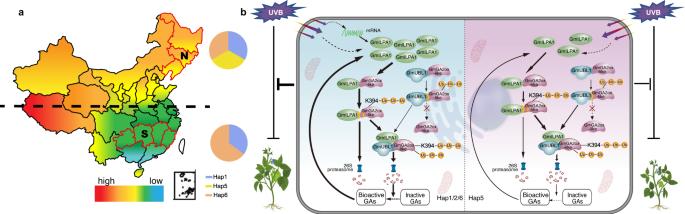Fig. 8: A working model of the regulation of plant height by the GmILPA1-GmUBL1-GmGA2ox-like module in soybean. aGeographical distribution ofHap1,Hap5andHap6. N, north of China, S, south of China. The pie chart represents their frequency.bThe working model of GmILPA1 regulating of plant height inHap1/2/6andHap5. InHap1/2/6, under the UV-B irradiation, GmILPA1 accumulation is induced at transcriptional and protein levels. GmGA2ox-like is ubiquitinated by GmILPA1 and GmUBL1, and GmILPA1 mediates the degradation of GmGA2ox-like, GmUBL1 enhanced the degradation of GmGA2ox-like. As a result, the increase of bioactive GAs content promoted the growth of soybean. InHap5, under the UV-B irradiation, GmILPA1 accumulation is induced only at protein level, eventually leads to shorter plant height inHap5. GA3 induces GmILPA1 protein accumulation both inHap1/2/6andHap5. Phylogenetic analysis was based on UPGMA tree implemented in MEGA7 software. Detection of selection signals, nucleotide diversity, and tests for neutrality The fixation index (FST), nucleotide diversity, and Tajima’s D values in wild, landrace, and cultivated soybean germplasms were calculated across the ~3.7-kb genomic region of GmILPA1 that includes the ~2.0-kb promoter, exons, introns, and 5′ and 3′ UTR sequences under a 100-kb sliding window analysis with a 5-kb step using VCFtools (v0.1.14). β-Glucuronidase (GUS) assay The GmILPA1pro Hap1 :GUS , GmILPA1pro Hap3 :GUS , GmILPA1pro Hap5 :GUS , GmILPA1pro Hap5/indel :GUS and GmILPA1pro Hap6 :GUS reporter constructs were independently transformed into Agrobacterium strain GV3101 for transient expression via Agrobacterium -mediated infiltration. The plants were incubated for 3 days at 25 °C. For UV-B treatment, the plants were treated with UV-B for 12 h before the infiltrated leaves were collected. N. benthamiana leaf discs were stained with 5-bromo-4-chloro-3-indolyl β-D-glucuronide (X-Gluc) for 24 h at 37 °C. For measurements of GUS activity, 4-methylumbelliferyl β-D-glucuronide (4-MUG) was added as substrate for a fluorometric assay, and the amount of 4-MU produced in the GUS reaction was measured on a Thermo Scientific Microplate Reader (Thermo Scientific). The total concentration of protein extracted from the leaf discs was measured using a BCA Protein Assay (Thermo Scientific) and diluted to a reaction concentration of 50 μg ml –1 . Final GUS activity was calculated according to a standard curve of 4-MU and expressed as pmol 4-MU/μg /min. The GUS assays were performed three times. Enzyme activity of recombinant GmGA2ox-like protein The full-length cDNAs of GmGA2ox-like were cloned into the pEGX4T-2 vector. Construct was confirmed and transformed into Escherichia coli Transetta (DE3) (Transgene) for recombinant protein expression. The pEGX4T-2 vector was used as a control. For the enzyme activity assay, the procedure was adapted from previous studies with slight modification [81] , [82] . One hundred micrograms of total protein was incubated with GA metabolites (1 μg) in 100 μl of reaction mixture containing 100 mM Tris–HCl (pH 7.5), 1 mM FeSO4, 10 mM 2-oxoglutarate, 10 mM ascorbate, and 5 mM DTT at 30 °C for up to 6 h. After incubation, 100 μl of methanol was added and mixed. After centrifugation the supernatant was collected for analysis by LC–MS/MS (AB SECIEX API5500). A C18 HPLC capillary column (Agilent, 100 mm × 2.1 mm × 2.7 μm) was used for separation. Mobile phase was composed of solvent A (0.1% formic acid) and solvent B (100% MeOH). Solvent gradient was programmed as 15% of solvent B for 2 min, increasing solvent B to 95% over 15 min, holding for 3 min, and returning back to 5% of solvent B over 2 min, followed by a 5-min re-equilibration prior to the next sample injection. Flow rate was maintained at 0.3 ml/min. Each sample injection volume was 50 μl. MS spectra were acquired in negative electrospray ionization combined with the SRM (selected-reaction monitoring) mode and analyzed using software (Analyst). Statistics and reproducibility Significant differences were analysed using two-sample Student’s t -tests or one-way ANOVA with GraphPad Prism 8.0. All experiments were repeated independently three times. Reporting summary Further information on research design is available in the Nature Portfolio Reporting Summary linked to this article.